Validation of climate model-inferred regional temperature change for late-glacial Europe Comparisons of climate model hindcasts with independent proxy data are essential for assessing model performance in non-analogue situations. However, standardized palaeoclimate data sets for assessing the spatial pattern of past climatic change across continents are lacking for some of the most dynamic episodes of Earth’s recent past. Here we present a new chironomid-based palaeotemperature dataset designed to assess climate model hindcasts of regional summer temperature change in Europe during the late-glacial and early Holocene. Latitudinal and longitudinal patterns of inferred temperature change are in excellent agreement with simulations by the ECHAM-4 model, implying that atmospheric general circulation models like ECHAM-4 can successfully predict regionally diverging temperature trends in Europe, even when conditions differ significantly from present. However, ECHAM-4 infers larger amplitudes of change and higher temperatures during warm phases than our palaeotemperature estimates, suggesting that this and similar models may overestimate past and potentially also future summer temperature changes in Europe. The late-glacial period ~15–11 thousand years ago (ka BP) was characterized by major changes in climate forcings such as the extent of ice sheets, atmospheric greenhouse gas concentrations and ocean circulation [1] , [2] , [3] , [4] . The North Atlantic region experienced abrupt variations in climate during this period, including rapid warming phases at the beginning of the Bølling–Allerød Interstadial (BA-IS) at ~14.6 ka BP and the Holocene at ~11.7 ka BP, and abrupt cooling at the beginning of the Younger Dryas (YD) at ~12.7 ka BP [4] , [5] , [6] , [7] . Since these climatic changes were driven by processes that are also expected to play an important role in determining future climate, for example variations in ocean circulation and atmospheric greenhouse gas concentrations, this period provides a crucial time interval for understanding the response of the global climate system to rapid changes in climate forcings, and for testing climate model simulations under strongly varying boundary conditions [1] , [8] , [9] , [10] . To evaluate model performance against climate reconstructions, large and geographically extensive data sets are required that encompass regional temperature patterns. Such data sets are particularly relevant for demonstrating that climate models can adequately predict regionally diverging trends in climatic change, since the spatial resolution of most climate models presently allows for only coarse representation of geographical and topographic features important for regional climates (for example, complex coastlines or mountain chains). Available temperature reconstructions from Europe are based on different approaches and protocols, and include proxy types that are not only affected by temperature, but also strongly influenced by precipitation and effective moisture [11] , [12] . Hence, it is difficult to assess whether variations in temperature development reconstructed for different regions are a consequence of different proxy types and methodologies, confounding climatic variables or varying temperature gradients across the continent. To resolve this, standardized data sets are necessary, based on proxy indicators that consistently reflect temperature and are influenced to a lesser extent by changing precipitation or moisture. Furthermore, reconstructions should be based on a consistent and quantitative numerical approach that provides estimates of mean climate states rather than temperature ranges as are provided by some approaches to climate reconstruction. Here we use fossil assemblages of chironomid larvae (non-biting midges) preserved in lake sediments to reconstruct variations in summer temperature across Europe. Chironomid larvae are aquatic, and in lakes, winter ice-cover decouples their habitat from the direct influence of sub-zero temperatures. Therefore, chironomid assemblages are less strongly influenced by winter temperature than many other biotic temperature indicators [13] , [14] . The occurrence and abundance of chironomids in lakes are closely related to summer air and water temperatures allowing summer temperature to be estimated from chironomid assemblages [14] , [15] . In lakes, chironomid distribution is affected by water depth [16] , [17] , and therefore hydrological changes may influence chironomid assemblage composition if they lead to major changes in the water level. However, in the shallow lake basins that are commonly used for temperature reconstruction, changes in water depth have only a relatively minor influence on chironomid-inferred temperatures [17] as long as they do not lead to a drying out or salinization of the lake. Chironomids have previously been used to reconstruct regional variations in temperatures in northeastern North America [18] and northwest Europe [19] . However, detailed reconstructions of latitudinal and longitudinal temperature gradients across continents have not yet been attempted. We present palaeotemperatures reconstructed from 31 fossil chironomid sequences in Europe, covering parts of or the entire period 15–11 ka BP ( Fig. 1 ) (see Methods). Stacked and spliced reconstructions of regional temperatures have been compiled based on the available complete or fragmentary records to summarize past July air temperature changes across the continent. We compare our chironomid-based temperature reconstructions with hindcasts of regional changes in summer temperature across Europe produced by the ECHAM-4 Atmospheric General Circulation Model [1] . Though more recent versions of the ECHAM model are now available (ECHAM-5–6), these hindcasts still provide the spatially most explicit late-glacial climate model runs for Europe. We show that regional patterns of temperature change reconstructed by our new chironomid-based data set are in excellent agreement with summer temperature changes inferred across Europe by ECHAM-4, confirming that such models can correctly predict regional changes in summer temperature across the continent in periods when climate boundary conditions were substantially different from present. However, the model reconstructs larger amplitudes of change and higher temperatures during warmer climatic phases than indicated by our chironomid-based estimates. 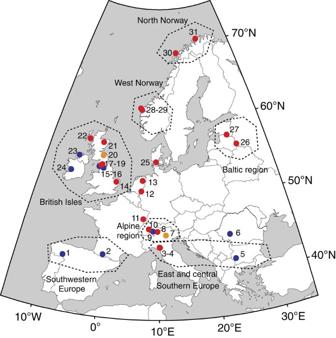Figure 1: Location of the chironomid-based temperature records in Europe. Site numbers are explained inSupplementary Table 1. Records cover the YD/EH transition (red), ELG/BA-IS transition (orange) or both (blue). Dotted lines indicate the regions for which stacked records are provided inFig. 2. Figure 1: Location of the chironomid-based temperature records in Europe. Site numbers are explained in Supplementary Table 1 . Records cover the YD/EH transition (red), ELG/BA-IS transition (orange) or both (blue). Dotted lines indicate the regions for which stacked records are provided in Fig. 2 . Full size image Geographical pattern of temperature change All the major climatic transitions in the interval studied at ~14.6, ~12.7 and ~11.7 ka BP are apparent in the stacked reconstructions ( Fig. 2 ). At similar latitudes, chironomid-inferred temperature variations tend to be most pronounced in western Europe (British Isles, southwestern Europe) and more muted in the east (central and southeastern sectors, Fig. 2 ). Stacked records from western Europe and the Baltic indicate that temperatures during the early Holocene (EH) were similar to those during the BA-IS ( Fig. 2 ). Elsewhere, EH temperatures were warmer than during the BA-IS. We compared latitudinal temperature gradients across Europe for the time slices ~11.4, ~12.0, ~13.0, ~14.45 and ~14.9 ka BP, representing the EH, YD, late BA-IS, early BA-IS and early late-glacial just preceding the BA-IS (ELG), respectively ( Fig. 3 ). EH temperatures ( Fig. 3a ) were overall slightly cooler than today, but showed a similar latitudinal summer temperature gradient to that at present (~0.5 °C per degree latitude). EH and BA-IS ( Fig. 3c,d ) latitudinal temperature gradients resembled each other, although in the BA-IS, temperatures were slightly lower than in the EH, especially to the north. YD summer temperatures were characterized by a very steep temperature gradient ~48–53°N ( Fig. 3b ). Temperatures were, on average, 5.9 °C below present values north of 52°N, but only 3.5 °C lower south of 52°N. ELG temperatures north of ~52°N were similar to YD temperatures (average difference 0.2 °C, Fig. 3f ). To the south, ELG temperatures were clearly lower than YD temperatures (average difference 2.6 °C). Reconstructed temperatures in the early BA-IS were cooler than in the late BA-IS east of 10°E, but similar to or higher than late BA-IS temperatures west of 10°E ( Fig. 4 ). 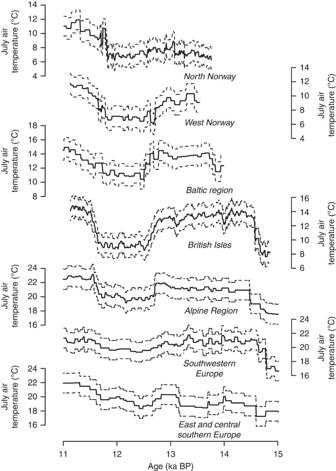Figure 2: Regional temperature reconstructions for different parts of Europe. Stacked and spliced July temperature reconstructions were calculated based on the individual chironomid-inferred temperature records available for different regions of Europe. Dashed lines indicate the estimated error of prediction (see Methods). Inferred temperatures are adjusted to modern sea level. Ages are indicated as thousands of calendar years (ka) before present (0 ka BP=1950 AD). Figure 2: Regional temperature reconstructions for different parts of Europe. Stacked and spliced July temperature reconstructions were calculated based on the individual chironomid-inferred temperature records available for different regions of Europe. Dashed lines indicate the estimated error of prediction (see Methods). Inferred temperatures are adjusted to modern sea level. Ages are indicated as thousands of calendar years (ka) before present (0 ka BP=1950 AD). 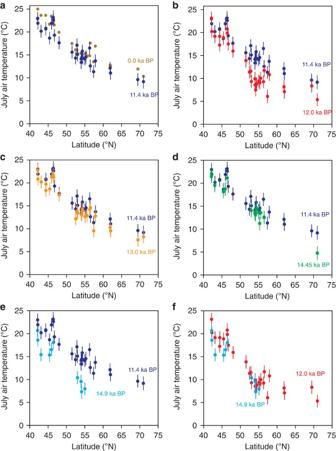Figure 3: Latitudinal changes in July temperature across Europe. (a) EH (~11.4 ka BP, dark blue) compared with modern temperatures (brown); (b) EH compared with YD (~12.0 ka BP, red); (c) EH compared with late BA-IS (~13.0 ka BP, orange); (d) EH compared with early BA-IS (~14.45 ka BP, green); (e) EH compared with ELG (~14.9 ka BP, light blue); (f) YD compared with ELG. Inferred temperatures are adjusted to modern sea level. Full size image Figure 3: Latitudinal changes in July temperature across Europe. ( a ) EH (~11.4 ka BP, dark blue) compared with modern temperatures (brown); ( b ) EH compared with YD (~12.0 ka BP, red); ( c ) EH compared with late BA-IS (~13.0 ka BP, orange); ( d ) EH compared with early BA-IS (~14.45 ka BP, green); ( e ) EH compared with ELG (~14.9 ka BP, light blue); ( f ) YD compared with ELG. Inferred temperatures are adjusted to modern sea level. 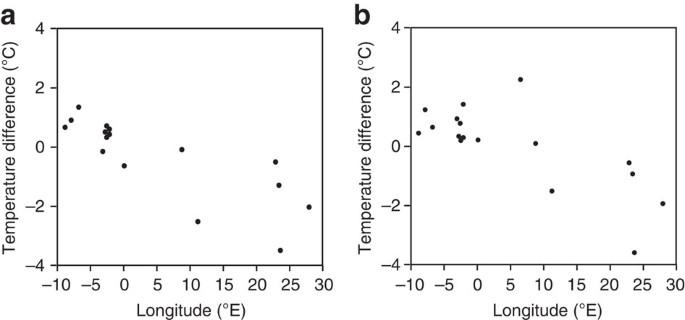Figure 4: Temperature trends within the BA-IS. Differences between July temperatures reconstructed by the chironomid records for the early BA-IS and the late BA-IS are plotted relative to longitude. Differences are shown between the periods ~14.45 and ~13.0 ka BP (a) and ~14.25 and ~13.0 ka BP (b). Full size image Figure 4: Temperature trends within the BA-IS. Differences between July temperatures reconstructed by the chironomid records for the early BA-IS and the late BA-IS are plotted relative to longitude. Differences are shown between the periods ~14.45 and ~13.0 ka BP ( a ) and ~14.25 and ~13.0 ka BP ( b ). Full size image Comparison with ECHAM-4 runs ECHAM-4 climate model runs available for the late-glacial simulate major variations in the amplitude of warming at the beginning of the BA-IS and the EH across Europe ( Fig. 5 ). In the model, warming at both transitions is largely forced by changes in North Atlantic overturning, and the most pronounced temperature increase is recorded at mid-latitudes (50–60°N). The influence of these variations in ocean circulation is dampened farther inland, resulting in a distinct west–east gradient in the amplitude of warming in Europe. Chironomid-based reconstructions confirm these regional climatic patterns. The amplitude of warming at the beginning of the BA-IS decreases across the continent from west to east in both proxy and model results ( Fig. 5a ). Latitudinal variations in amplitude are also very similar for both approaches, although for the ELG/BA-IS transition climatic changes in northern Europe are not adequately represented in our proxy data due to an absence of records >56°N. For the EH warming, the strongest temperature increases are inferred by both approaches at ~53–60°N ( Fig. 5b ). Although relative temperature changes are very similar in both model and proxy results, temperature variations simulated by ECHAM-4 are generally of higher amplitude than those inferred from chironomids ( Fig. 5a,b ). A comparison of absolute July temperature estimates at each site reveals that the largest offsets between the two approaches are found for grid cells that were considered to be still covered by continental ice sheets in the model ( Fig. 5c ). For these locations, the spatial resolution of ECHAM-4 is not sufficient to resolve fine-scale dynamics of continental ice retreat, leading to the prediction of ice masses at locations in which lakes already existed. For sites unaffected by ice-sheet dynamics, model- and proxy-based estimates are closely correlated ( Fig. 5c ). However, estimates provided by ECHAM-4 are distinctly higher than proxy-based temperatures during the warm phases (BA-IS, EH), suggesting that ECHAM-4 may be overestimating July temperatures during warmer climatic conditions of the late-glacial period compared with chironomid-inferred reconstructions. 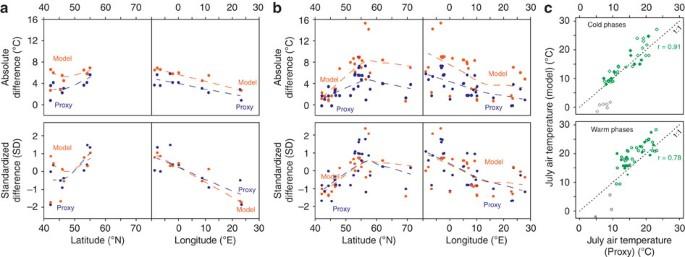Figure 5: Comparison of proxy-based temperature estimates with climate model runs. Chironomid-inferred July temperatures are compared with July temperatures as hindcast for our sites by the ECHAM-4 climate model1. (a,b) Latitudinal and longitudinal variations in absolute and standardized temperature changes for the ELG/BA-IS (a) and YD/EH transition (b). (c) Direct comparison of chironomid- and model-inferred July temperatures for the cold (upper panel) and warm phases (lower panel) of the examined time interval (open diamonds: YD, filled diamonds: ELG, open circles: EH, filled circles: BA-IS). Sites in grid cells for which the model assumes the presence of continental ice sheets are plotted in grey (not taken into account for calculating Pearson correlation (r) values). Dashed lines ina,bare fitted using locally weighted regression (LOESS) (span 1.0). Dashed lines increpresent unity. Figure 5: Comparison of proxy-based temperature estimates with climate model runs. Chironomid-inferred July temperatures are compared with July temperatures as hindcast for our sites by the ECHAM-4 climate model [1] . ( a , b ) Latitudinal and longitudinal variations in absolute and standardized temperature changes for the ELG/BA-IS ( a ) and YD/EH transition ( b ). ( c ) Direct comparison of chironomid- and model-inferred July temperatures for the cold (upper panel) and warm phases (lower panel) of the examined time interval (open diamonds: YD, filled diamonds: ELG, open circles: EH, filled circles: BA-IS). Sites in grid cells for which the model assumes the presence of continental ice sheets are plotted in grey (not taken into account for calculating Pearson correlation ( r ) values). Dashed lines in a , b are fitted using locally weighted regression (LOESS) (span 1.0). Dashed lines in c represent unity. Full size image The excellent agreement of the geographical pattern of warming at the ELG/BA-IS and YD/EH transitions in both ECHAM-4 and our new proxy data set impressively confirms that the climatic-forcing mechanisms assumed to lead to changes in temperature gradients across Europe in the model are likely to be correct. Increasing summer insolation caused progressively warmer summers with increasing distance from the North Atlantic. Changes in the North Atlantic overturning [2] , [20] and associated latitudinal shifts in sea ice [1] were responsible for the large amplitude of summer temperature changes along the Atlantic seaboard 52–60°N. Cooler ELG than YD temperatures in southern and central Europe can be explained by the more southerly position of North Atlantic sea-ice during the ELG [21] . Finally, long-term temperature changes observed during the BA-IS suggest that, along the North Atlantic seaboard south of 65°N, enhanced North Atlantic overturning circulation [22] led to warmer temperatures early in the BA-IS, whereas farther away from the Atlantic, summer temperatures followed the long-term summer insolation trend ( Fig. 4 ). Chironomid-based palaeotemperature estimates reproduce the geographical pattern of past summer temperature change predicted in the ECHAM-4 runs ( Fig. 5 ). Earlier comparisons of these model runs with summer temperature proxy data were based on minimum estimates of mean July temperature calculated from the occurrence of temperature-sensitive plant species in different parts of northwest Europe [1] . This provided support for distinct latitudinal summer temperature gradients across Europe during the late-glacial period, as inferred by ECHAM-4. However, such minimum estimates of mean July temperature are of only limited use for direct proxy-to-climate model comparisons, since any temperature prediction higher than the reconstructed minimum temperature estimate will be in agreement with the proxy data. Furthermore, differences in minimum temperature estimates based on plant occurrences calculated for different periods in the past are not necessarily expected to reflect past differences in mean temperatures. In contrast, our mean temperatures reconstructed from chironomid assemblages can be directly plotted against mean temperatures inferred by ECHAM-4 ( Fig. 5c ) and provide support for both the latitudinal differences in the amplitude of late-glacial temperature changes inferred by ECHAM-4 across Europe, and the longitudinal ones ( Fig. 5a,b ). Our palaeotemperature-climate model comparison ( Fig. 5 ) confirms that general circulation models, such as ECHAM-4, can correctly predict regionally varying temperature changes across Europe in periods when climate-forcing mechanisms were substantially different from present, assuming that realistic boundary conditions are prescribed. At the same time, the smaller amplitudes of variations inferred by chironomid records suggest that climate reconstructions by ECHAM-4 and similar models may be overestimating European summer temperature change during the late-glacial and EH. The most pronounced divergence is observed for high latitudes during the YD/EH transition ( Fig. 5 ). This raises the possibility that future climate changes associated with variations in forcing factors that were dominant in the late-glacial and EH period (for example, North Atlantic circulation, greenhouse gas concentrations) may also be overestimated by models such as ECHAM-4. Further, independent proxy-based estimates of variations in past temperatures across Europe at similar spatial coverage as our data, and additional hindcasts of late-glacial and EH climates with the newest generation of climate models will ultimately be needed to resolve this discrepancy between model and proxy results. Lake sediment records The examined lake sediment sequences were obtained from small lacustrine basins, similar in size to those used for developing the applied chironomid-temperature transfer function [23] . They span a geographical range of 42–71°N and 9°W–28°E ( Supplementary Table 1 ). The sequences contain part of or the entire interval 15–11 ka BP and have been dated using a range of approaches, including 14 C dating of terrestrial plant remains, tephrochronology and correlation to other well-dated sequences using palynostratigraphy, lithostratigraphy or isotope stratigraphical methods ( δ 18 O analysed on lake marl). Absolute dating of late-glacial sediment sequences is challenging due to several radiocarbon plateaux during the late-glacial, a low number of dateable terrestrial plant remains deposited in the unforested landscapes that covered large sections of Europe, and the frequent occurrence of disturbances in the lakes and their catchment (for example, vegetation change, associated changes in erosion, lake-level fluctuations) leading to mobilization and redeposition of terrestrial organic matter. As a consequence, we expect relatively large errors in the absolute dating (up to several centuries) for most records. However, our records are well constrained stratigraphically (for example, via pollen or isotope analysis), allowing the determination of the major stratigraphic and climatological units of the late-glacial. These include the ELG (>14.7 ka BP) preceding the BA-IS, the Bølling and Allerød biozones, together forming the BA-IS (14.6–12.7 ka BP), the YD cool period (12.7–11.7 ka BP) and the EH (<11.7 ka BP). As a consequence, the time intervals discussed here, including the examined time slices of ~11.4, ~12.0, ~13.0, ~14.25, ~14.45 and ~14.9 ka BP, representing the EH, the YD, the late Allerød, the middle-to-late Bølling, the early Bølling and the ELG, respectively, are well constrained in our data. To ensure a consistent chronological approach for all records, ages were assigned to individual samples based on linear interpolation between dated horizons. In cases where this was considered feasible, ages were extrapolated beyond the oldest/youngest chronological marker to include sections of the records just preceding or after the usually well-constrained climatic transitions of the late-glacial. Extrapolations are based on the sedimentation rates of adjacent sediment sections. In all cases extrapolations do not exceed 500 years. In a few records, age markers are based on the major changes of chironomid-inferred temperatures at the YD/EH and ELG/BA-IS transitions ( Supplementary Table 2 ). Where these events are used as chronological constraints, either as identified in the chironomid records, or as determined by independent stratigraphical methods (for example, palynostratigraphy, δ 18 O), we used estimates for the age of these climatic transitions (the period of maximum change) as determined from the NGRIP δ 18 O record [24] . The resulting ages are 14.64 ka BP for the ELG/BA-IS transition (in Greenland equivalent to the Greenland Stadial (GS)-2/Greenland Interstadial (GI)-1 transition), 12.71 ka BP for the BA-IS/YD transition (GI-1/GS-1 transition) and 11.63 ka BP for the YD/EH transition (GS-1/Holocene transition). All ages are given as thousands of calendar years (ka) before present, where 0 ka BP is equivalent to 1950 AD. Radiocarbon-based age estimates have been converted to calibrated radiocarbon ages BP (cal. BP). However, since our age determinations include both radiocarbon dating and nonradiocarbon approaches, ages are reported as ka BP instead of ka cal. BP. The sediment sequences have been obtained by a range of coring methods and in one case from an exposed sediment profile. With the exception of several new records from southern, eastern, central and northern Europe, the records are described in a number of site-specific publications ( Supplementary Table 1 ). Chironomid-based temperature reconstructions All chironomid records were produced using standardized methods [25] , and chironomid taxa were identified by the two principal analysts (O.H., S.J.B.) or scientists trained by them. Taxonomy followed the descriptions in ref. 25 . July air temperature reconstruction based on fossil chironomid assemblages was implemented using a modern chironomid-temperature calibration data set consisting of chironomid assemblage data and mean July air temperature values for 274 lakes in Norway and Switzerland [23] . A transfer function for reconstructing mean July air temperature based on fossil chironomid assemblages was developed from the calibration data using weighted-averaging partial least-squares regression [26] , [27] and the software C2 (ref. 28 ). During model development, 19 of the calibration data set lakes were deleted as outliers [23] . Error statistics for this model were estimated using 9999 bootstrapping cycles. At the highest taxonomic resolution, the inference model predicted mean July air temperature in the modern calibration data with a root mean square error of prediction of 1.40 °C and a coefficient of determination between inferred and observed July air temperature values of 0.87 ( Supplementary Table 2 ). For a number of records, several fossil types had to be amalgamated into single-taxonomic categories, either because poor preservation of the fossil remains did not allow reliable separation of some morphotypes or, in a few cases, because the identification of the assemblages took place before certain fossil chironomid taxa had been segregated. As a consequence, there are slight differences in the taxonomic resolution of the records and the applied transfer functions ( Supplementary Table 2 ). However, these differences are minor. A total of 151 taxa is included in the transfer function with the highest taxonomic resolution and 133 taxa in the model with the lowest resolution. Taxonomic differences of this scale have only minor effects on chironomid-based temperature inferences [29] . Modern temperature data and elevational correction Modern temperature data were obtained from the New et al . [30] climatology. For comparison with fossil records, mean July air temperatures for the closest grid cells to the study site were extracted from the data set. All temperatures—modern and chironomid-inferred—were corrected to 0 m asl using a modern July air temperature lapse rate of 6 °C km −1 (refs 31 , 32 ). All chironomid-inferred July air temperature values were within the temperature range encompassed by the calibration data set (3.5–18.4 °C) before elevational correction. Screening and outlier deletion Within the dated interval, chironomid-based temperature records were screened for unusual values leading to the deletion of seven out of a total of 1,431 chironomid-inferred temperature values. In some records, chironomid-inferred temperatures or the stratigraphic integrity of the sediment record were considered unreliable. These sections were excluded from further analysis leading to a deletion of a further 18 samples. Of these, 13 originated from the site Lusvatnet, for which pollen analysis indicated contaminated sediments for a section of the record, two are from the site Slotseng and contain invertebrate and plant assemblages that indicate drying up of the lake basin, and three originate from the site Lago di Lavarone and were based on a very low count size (see Supplementary Table 2 and references in Supplementary Table 1 ). Stacking and splicing Individual chironomid records can be affected by site-specific factors (for example, aspect, groundwater or running water influence). Furthermore, many of the chironomid records were fragmentary, covering only parts of the late-glacial. Therefore, stacked records, based on several (usually 2–4) records, were produced to summarize temperature trends for different regions of Europe ( Fig. 2 ). The procedure used to develop these regional reconstructions is summarized graphically in Supplementary Fig. 1 . Stacks were produced by interpolating reconstructed temperatures to constant time intervals (10 years) using the nearest neighbour algorithm for calculating interpolated values. Averages of several records then provided stacked records for July air temperature for a particular time interval and region. Few of the chironomid records were continuous over the entire time window of interest. Therefore, different sections of the stacks were usually based on a variable number of records ( Supplementary Fig. 2 ). Since some of the records tended to reconstruct cooler or warmer temperatures than others—a tendency related to the relative geographical position of the sites or to other site-specific factors—the absence of data from a particular site can have a noticeable effect on the mean temperatures in a stack. To correct for this, we produced several stacked records for regions with fragmentary temporal coverage of the late-glacial, with each stack based on the temperatures from the same subgroup of localities. These stacks were calculated so that there was an overlap with younger/older stacked records, which allowed the calculation of offsets between the different stacks. This, in turn, allowed a correction (‘splicing’) of the individual stacked records to produce continuous regional reconstructions unaffected by local site-specific effects. The spliced records were anchored to the stack based on the highest number of chironomid records. Overlaps between stacks were chosen to be between 500 and 1,000 years, depending on the variability and similarity of the different stacked temperature records. Variations in the resulting stacked and spliced records are driven by changes in the individual chironomid-based temperature reconstructions, whereas the absolute value is determined by the average temperatures of the section based on most chironomid records (the ‘anchoring’ section). Splicing of stacks works best for relatively long, continuous records, since this allows long sections of overlap between individual stacked records. Also, a large number of splices increases the likelihood of artefacts in the regional reconstructions. We therefore limited the number of records included in any given stacked section to four, even in regions and for time intervals for which more chironomid records would have been available. In these instances, records were selected based on the quality of the chronological data, the length of the records and their sampling resolution. Estimated standard errors of prediction for the stacks were calculated as the square root of the average of the squared sample-specific errors of the individual palaeotemperature records used to produce the stacks. This error estimate represents the uncertainty of transforming chironomid assemblage data to quantitative temperature inferences based on the transfer function and of combining multiple reconstructions into a single ‘stacked’ temperature estimate. It does not represent uncertainties in the reconstructed July air temperatures associated with dating and interpolating the individual reconstructions. ECHAM-4 model runs The ECHAM-4 model runs presented in Fig. 5 have been described in detail elsewhere [1] . They are based on the T42 version of the model (spatial resolution of ~2.8° × 2.8° latitude/longitude). The four model runs we discuss, representing climate conditions during the GS-2a, GI-1e, GS-1 and the Preboreal, were performed by changing boundary conditions (ocean surface conditions, ice sheets, insolation, greenhouse gas concentrations, vegetation) to represent these time intervals. Differences in July air temperature between GS-2a and GI-1e and between GS-1 and the Preboreal represent modelled changes at the ELG/BA-IS and YD/EH transition, respectively, and are plotted versus our chironomid-inferred temperature differences in Fig. 5 . How to cite this article : Heiri, O. et al . Validation of climate model-inferred regional temperature change for late-glacial Europe. Nat. Commun. 5:4914 doi: 10.1038/ncomms5914 (2014).